Collagen VI regulates satellite cell self-renewal and muscle regeneration Adult muscle stem cells, or satellite cells have essential roles in homeostasis and regeneration of skeletal muscles. Satellite cells are located within a niche that includes myofibers and extracellular matrix. The function of specific extracellular matrix molecules in regulating SCs is poorly understood. Here, we show that the extracellular matrix protein collagen VI is a key component of the satellite cell niche. Lack of collagen VI in Col6a1 –/– mice causes impaired muscle regeneration and reduced satellite cell self-renewal capability after injury. Collagen VI null muscles display significant decrease of stiffness, which is able to compromise the in vitro and in vivo activity of wild-type satellite cells. When collagen VI is reinstated in vivo by grafting wild-type fibroblasts, the biomechanical properties of Col6a1 –/– muscles are ameliorated and satellite cell defects rescued. Our findings establish a critical role for an extracellular matrix molecule in satellite cell self-renewal and open new venues for therapies of collagen VI-related muscle diseases. Interactions between cells and extracellular matrix (ECM) have key roles in tissues undergoing extensive mechanical stress, such as skeletal muscles [1] . A major component of the ECM of skeletal muscles is collagen VI, a protein composed by three genetically distinct chains and forming a discrete network of beaded microfilaments in the basement membrane of muscle endomysium [2] , [3] . Collagen VI deposition in skeletal muscles is mainly provided by interstitial muscular fibroblasts [4] . Moreover, expression of collagen VI genes is regulated by myogenic cells, whose presence is a prerequisite for inducing the deposition of collagen VI by fibroblasts [5] . The critical role of collagen VI in skeletal muscles is supported by the fact that mutations of COL6 genes in humans cause various muscle disorders, including Bethlem myopathy and Ullrich congenital muscular dystrophy [2] , [3] . Collagen VI null ( Col6a1 –/– ) mice display a mild myopathic phenotype associated with mitochondrial dysfunction, defective autophagy and spontaneous apoptosis of muscle fibers [6] , [7] , [8] . Satellite cells (SCs) are located between the basal lamina and the plasma membrane of muscle fibers [9] , and this anatomic localization represents their niche. This niche is characterized by an asymmetric distribution of muscle components, where SCs contact myofibers through the apical surface whereas the ECM lies on their basal surface [9] , [10] . The myogenic commitment and differentiation of SCs is under the control of key transcription factors, such as the paired box protein 7 (Pax7) and the myogenic regulatory factors MyoD and Myogenin (MyoG) [11] , [12] , [13] , [14] , [15] . During muscle regeneration, SCs undergo proliferation, generating both a stem cell population by self-renewal and more differentiated cells that give rise to myoblasts that undergo terminal differentiation and fusion [16] . A growing body of evidence indicates that the niche serves as an instructive environment by which SCs respond to extrinsic stimuli associated with muscle growth and repair [17] , [18] , [19] , [20] , [21] , [22] , [23] . Changes in the ECM composition provide regulatory cues to SCs, thus influencing their quiescence, activation, differentiation and/or self-renewal [24] . On the other hand, ECM composition affects the mechanical properties of tissue microenvironment, which in turn influence the activity of various stem cells, including SCs [25] , [26] . Here, we demonstrate that collagen VI is a critical component of SC niche that is required for preserving SC self-renewal and muscle regeneration. In vitro and in vivo data indicate that one key mechanism through which collagen VI regulates SC activity is the modulation of muscle stiffness. Grafting with wild-type fibroblasts elicits extensive deposition of collagen VI and rescues SC self-renewal and muscle stiffness in Col6a1 –/– mice. Our findings provide novel insights into the relevance of collagen VI for skeletal muscles and reveal an unforeseen role for this ECM molecule in the regulation of SC homeostasis. Collagen VI is an extracellular component of SC niche We first evaluated collagen VI synthesis and localization with respect to SCs in murine extensor digitorum longus (EDL) and tibialis anterior (TA) muscles. Collagen VI was abundant in the endomysium of both muscles, and the protein was adjacent to the surface of SCs ( Fig. 1a and Supplementary Fig. S1a ). The localization was also confirmed ex vivo on freshly isolated myofibers and on sorted SCs ( Fig. 1b ; Supplementary Fig. S1b,c and Supplementary Movies ). Interestingly, collagen VI was expressed by sorted SCs, and Col6a1 transcripts were regulated during SC activation. Differently from collagen I (the major collagen of muscle interstitial ECM), Col6a1 transcripts were abundant in quiescent SCs and their amount decreased in activated SCs ( Fig. 1c and Supplementary Table S1 ). When TA muscles were subjected to injury with cardiotoxin [27] , collagen VI deposition was markedly increased during the initial phases of regeneration and the protein was found nearby all Pax7 + cells 4 days after injury ( Fig. 1d and Supplementary Figs. S1d and S2 ). These data indicate that collagen VI is expressed by SCs in a regulated manner and is an ECM component of the niche whose deposition is markedly increased upon muscle regeneration. 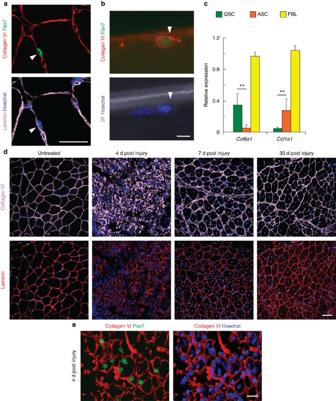Figure 1: Collagen VI is an extracellular component of SC niche. (a) Representative confocal image of immunofluorescence analysis for collagen VI (red), Pax7 (green) and laminin (light pink) in TA cross-sections from wild-type mice. The arrowhead points at one SC. Scale bar, 25 μm. (b) Representative confocal image of a freshly isolated wild-type EDL fiber, showing the immunolocalization of collagen VI (red) with respect to SC (green, arrowhead). BF, bright field. Scale bar, 10 μm. (c) Expression levels ofCol6a1andCol1a1transcripts in quiescent (QSC) and activated (ASC) wild-type SCs and in wild-type muscle fibroblasts (FBL).Gapdhexpression was used to calculate the relative expression ofCol6a1andCol1a1transcripts. Data are shown as mean±s.e.m. of three independent replicates (**P<0.01; unequal variance Student’st-test;n=8, each group). (d) Representative confocal z-stack images of immunofluorescence for collagen VI (light pink) and laminin (red) in TA cross-sections from wild-type mice under untreated conditions or 4 days, 7 days and 30 days after single cardiotoxin injury. Scale bar, 50 μm. (e) Representative views of immunofluorescence for collagen VI (red) and Pax7 (green) in wild-type TA 4 days after cardiotoxin injection. Nuclei were stained with Hoechst (blue). Scale bar, 50 μm. Figure 1: Collagen VI is an extracellular component of SC niche. ( a ) Representative confocal image of immunofluorescence analysis for collagen VI (red), Pax7 (green) and laminin (light pink) in TA cross-sections from wild-type mice. The arrowhead points at one SC. Scale bar, 25 μm. ( b ) Representative confocal image of a freshly isolated wild-type EDL fiber, showing the immunolocalization of collagen VI (red) with respect to SC (green, arrowhead). BF, bright field. Scale bar, 10 μm. ( c ) Expression levels of Col6a1 and Col1a1 transcripts in quiescent (QSC) and activated (ASC) wild-type SCs and in wild-type muscle fibroblasts (FBL). Gapdh expression was used to calculate the relative expression of Col6a1 and Col1a1 transcripts. Data are shown as mean±s.e.m. of three independent replicates (** P <0.01; unequal variance Student’s t -test; n =8, each group). ( d ) Representative confocal z-stack images of immunofluorescence for collagen VI (light pink) and laminin (red) in TA cross-sections from wild-type mice under untreated conditions or 4 days, 7 days and 30 days after single cardiotoxin injury. Scale bar, 50 μm. ( e ) Representative views of immunofluorescence for collagen VI (red) and Pax7 (green) in wild-type TA 4 days after cardiotoxin injection. Nuclei were stained with Hoechst (blue). Scale bar, 50 μm. Full size image Lack of collagen VI affects SCs and muscle regeneration Based on the above findings, we used collagen VI null ( Col6a1 –/– ) mice to explore the role of collagen VI in regulating SC function. In addition to abnormalities of muscle fibers in Col6a1 –/– mice (a higher incidence of centrally nucleated fibers and a lower mean myofiber cross-sectional area), there was an increased number of SCs, with a corresponding increase of SC proliferation and apoptosis, when compared with wild-type muscles ( Supplementary Figs. S3 and S4 ). We next subjected wild-type and Col6a1 –/– muscles to cardiotoxin injury. Despite the higher number of SCs before injury, Col6a1 –/– TA muscles displayed smaller newly forming myofibers 7 days after injury and the number of SCs between Col6a1 –/– and wild-type TA muscles was markedly reduced when compared with untreated animals ( Fig. 2a and Supplementary Fig. S5a ). To assess whether the observed alterations were simply due to delayed regeneration in Col6a1 –/– muscles, we analyzed TA 30 days after injury, when the late myogenic differentiation program was completed. Despite an increase of myofiber cross-sectional area, regenerated Col6a1 –/– muscles displayed a decreased number of SCs compared with untreated muscles ( Fig. 2b and Supplementary Fig. S5b ). These results indicate that lack of collagen VI leads to a decreased ability to properly maintain the SC pool after muscle damage, without any overt impairment of the differentiation and fusion of the SC progeny. To ascertain whether this phenotype was caused by a defective self-renewal ability of SCs, we performed multiple injury experiments and analyzed muscles 7 and 30 days after the last injury ( Supplementary Fig. S5c ). The inability of collagen VI-deficient muscles to regenerate properly after multiple rounds of injury was very evident. Following double injury, Col6a1 –/– TA muscles displayed a significantly lower number of newly forming myofibers 7 days after injury and a decrease of both myofiber cross-sectional area and muscle mass after 30 days ( Fig. 2c and Supplementary Fig. S5d,e ). This was even more striking in triple injury experiments, where muscle regeneration was dramatically impaired in Col6a1 –/– TA muscles, with extensive fibrotic lesions and significant decrease of muscle mass, while wild-type TA muscles were still able to regenerate properly ( Fig. 2c and Supplementary Fig. S5d,f ). Notably, following repeated injuries, Col6a1 –/– TA muscles showed a progressive decline in SC number ( Fig. 2e ). The progressive depletion of the SC pool in Col6a1 –/– muscles after injury indicates that collagen VI is strictly needed for the correct function of the niche and the maintenance of SC pool during muscle regeneration. 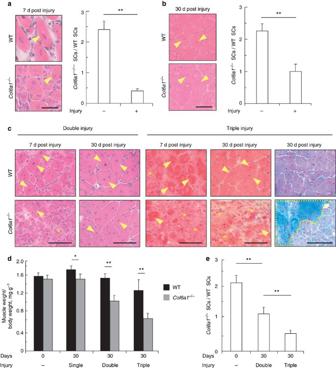Figure 2: Lack of collagen VI affects SC maintenance and muscle regenerationin vivo. (a) Left panel, haematoxylin-eosin staining of TA cross-sections from wild-type andCol6a1–/–mice 7 days after cardiotoxin injury. The arrowheads point at some newly forming myofibers. Scale bar, 25 μm. Right panel, ratio of SCs betweenCol6a1–/–and wild-type TA in untreated conditions (−) and 7 days after single injury (+). Data are shown as mean±s.e.m of three independent replicates (**P<0.01; unequal variance Student'st-test;n=6 animals, each group). (b) Left panel, haematoxylin-eosin staining of TA cross-sections from wild-type andCol6a1–/–mice 30 days after cardiotoxin injury. The arrowheads point at some newly forming myofibers. Scale bar, 50 μm. Right panel, ratio of SCs betweenCol6a1–/–and wild-type TA in untreated conditions (−) and 30 days after single injury (+). Data are shown as mean±s.e.m. of three independent replicates (**P<0.01; unequal variance Student’st-test;n=6 animals, each group). (c) Haematoxylin-eosin and Azan staining of TA cross-sections from wild-type andCol6a1–/–mice 7 days and 30 days after double and triple injury. Arrowheads point at some newly forming myofibers, asterisks label some areas still in the degeneration phase, and the dotted region in the lower right panel show fibrotic tissue substitution stained by Azan. Scale bar, 50 μm. (d) Quantification of TA weight/body weight of wild type andCol6a1–/–mice in untreated conditions (−) and 30 days after single, double or triple injury. Data are shown as mean±s.e.m. of three independent replicates (*P<0.05; **P<0.01; unequal variance Student’st-test;n=6–8 animals, each group). (e) Ratio of SCs betweenCol6a1–/–and wild-type TA in untreated conditions (−) and 30 days after double or triple injury. Data are shown as mean±s.e.m. of three independent replicates (**P<0.01; unequal variance Student’st-test;n=6 animals, each group). WT, wild-type. Figure 2: Lack of collagen VI affects SC maintenance and muscle regeneration in vivo . ( a ) Left panel, haematoxylin-eosin staining of TA cross-sections from wild-type and Col6a1 –/– mice 7 days after cardiotoxin injury. The arrowheads point at some newly forming myofibers. Scale bar, 25 μm. Right panel, ratio of SCs between Col6a1 –/– and wild-type TA in untreated conditions (−) and 7 days after single injury (+). Data are shown as mean±s.e.m of three independent replicates (** P <0.01; unequal variance Student's t -test; n =6 animals, each group). ( b ) Left panel, haematoxylin-eosin staining of TA cross-sections from wild-type and Col6a1 –/– mice 30 days after cardiotoxin injury. The arrowheads point at some newly forming myofibers. Scale bar, 50 μm. Right panel, ratio of SCs between Col6a1 –/– and wild-type TA in untreated conditions (−) and 30 days after single injury (+). Data are shown as mean±s.e.m. of three independent replicates (** P <0.01; unequal variance Student’s t -test; n =6 animals, each group). ( c ) Haematoxylin-eosin and Azan staining of TA cross-sections from wild-type and Col6a1 –/– mice 7 days and 30 days after double and triple injury. Arrowheads point at some newly forming myofibers, asterisks label some areas still in the degeneration phase, and the dotted region in the lower right panel show fibrotic tissue substitution stained by Azan. Scale bar, 50 μm. ( d ) Quantification of TA weight/body weight of wild type and Col6a1 –/– mice in untreated conditions (−) and 30 days after single, double or triple injury. Data are shown as mean±s.e.m. of three independent replicates (* P <0.05; ** P <0.01; unequal variance Student’s t -test; n =6–8 animals, each group). ( e ) Ratio of SCs between Col6a1 –/– and wild-type TA in untreated conditions (−) and 30 days after double or triple injury. Data are shown as mean±s.e.m. of three independent replicates (** P <0.01; unequal variance Student’s t -test; n =6 animals, each group). WT, wild-type. Full size image Collagen VI regulates SC activity in vitro Based on these results, we used different in vitro approaches to analyze the effects elicited by collagen VI on SCs. Sorted SCs were prepared from wild-type and Col6a1 –/– hindlimb muscles and cultured for 48 h on matrigel-coated dishes in the presence or absence of purified native collagen VI. To analyze the differentiation program, we divided cultured SCs into different populations. Early differentiation was evaluated on the basis of Pax7 and MyoD expression, by classifying cells in Pax7 + MyoD – , Pax7 + MyoD + and Pax7 – MyoD + populations [28] , whereas the onset of terminal differentiation was evaluated based on MyoG expression and by dividing cells into Pax7 + MyoG − and Pax7 − MyoG + populations [13] , [14] , [15] . When grown on matrigel, Col6a1 –/– cultures displayed lower percentages of Pax7-expressing cells and corresponding higher percentages of cells expressing MyoD or MyoG. By contrast, growth on collagen VI led to a significant increase of Pax7-expressing cells and decrease of differentiating cells in both wild-type and Col6a1 –/– cultures ( Supplementary Fig. S6a–c and Supplementary Tables S2 and S3 ). With the aim to reconstitute the ECM components found in the wild-type SC niche, we analyzed Col6a1 –/– single fibers cultured for 72 h on matrigel in the absence or presence of collagen VI. Col6a1 –/– SCs displayed a lower ability to preserve the Pax7 + MyoD − population in single fiber culture, as observed in SC-derived culture ( Fig. 3a and Table 1 ). When grown on dishes coated with purified collagen VI, Col6a1 –/– fibers contacted the collagen VI network, which also localized nearby SCs ( Fig. 3c and Supplementary Fig. S6d ). Remarkably, Col6a1 –/– SCs showed a higher ability to maintain the Pax7 + MyoD − population when fibers were grown on purified collagen VI, with decreased apoptosis and increased proliferation when compared with cultures grown on matrigel alone ( Fig. 3a ). Taken together, these in vitro data indicate that collagen VI improves the maintenance and survival of cells expressing Pax7, a transcription factor critical for SC self-renewal after damage [11] , [12] , [13] , [14] . 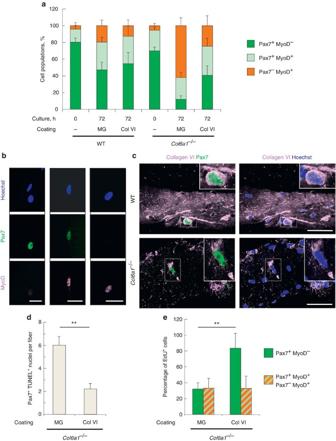Figure 3: Collagen VI regulates SC activityin vitro. (a) Quantification of Pax7+MyoD–, Pax7+MyoD+and Pax7–MyoD+cell populations on single wild-type andCol6a1–/–myofibers fixed upon isolation (0 h) or following 72 h culture on matrigel-coated dishes in the presence or absence of purified native collagen VI. Data are shown as mean±s.e.m. of three independent replicates. The statistical analysis is provided inTable 1(unequal variance Student’st-test;n=10–22 myofibers, each group). (b) Three representative confocal images of cultured single myofibers and labeled with antibodies for Pax7 (green) and MyoD (light pink). Nuclei were stained with Hoechst (blue). Scale bar, 20 μm. (c) Confocal z-stack images of wild-type andCol6a1–/–fibers grown on purified collagen VI and analyzed by immunofluorescence for collagen VI (light pink) and Pax7 (green). The insets show higher magnifications of the squared areas. Scale bar, 50 μm. (d) Quantification of apoptotic Pax7+cells by TUNEL test inCol6a1–/–single myofibers following 72 h culture on matrigel-coated dishes in the presence or absence of purified native collagen VI. Data are shown as mean±s.e.m. of two independent replicates (**P<0.01; unequal variance Student’st-test;n=10 myofibers, each group). (e) Quantification of EdU+cells, calculated as the percentage on Pax7+MyoD–, Pax7+MyoD+and Pax7–MyoD+cell populations, inCol6a1–/–single myofibers after 72 h culture on matrigel-coated dishes in the presence or absence of purified native collagen VI. Data are shown as mean±s.e.m. of three independent replicates (**P<0.01; unequal variance Student’st-test;n=10 myofibers, each group). Col VI, collagen VI; KO,Col6a1–/–; MG, matrigel; WT, wild-type. Figure 3: Collagen VI regulates SC activity in vitro . ( a ) Quantification of Pax7 + MyoD – , Pax7 + MyoD + and Pax7 – MyoD + cell populations on single wild-type and Col6a1 –/– myofibers fixed upon isolation (0 h) or following 72 h culture on matrigel-coated dishes in the presence or absence of purified native collagen VI. Data are shown as mean±s.e.m. of three independent replicates. The statistical analysis is provided in Table 1 (unequal variance Student’s t -test; n =10–22 myofibers, each group). ( b ) Three representative confocal images of cultured single myofibers and labeled with antibodies for Pax7 (green) and MyoD (light pink). Nuclei were stained with Hoechst (blue). Scale bar, 20 μm. ( c ) Confocal z-stack images of wild-type and Col6a1 –/– fibers grown on purified collagen VI and analyzed by immunofluorescence for collagen VI (light pink) and Pax7 (green). The insets show higher magnifications of the squared areas. Scale bar, 50 μm. ( d ) Quantification of apoptotic Pax7 + cells by TUNEL test in Col6a1 –/– single myofibers following 72 h culture on matrigel-coated dishes in the presence or absence of purified native collagen VI. Data are shown as mean±s.e.m. of two independent replicates (** P< 0.01; unequal variance Student’s t -test; n =10 myofibers, each group). ( e ) Quantification of EdU + cells, calculated as the percentage on Pax7 + MyoD – , Pax7 + MyoD + and Pax7 – MyoD + cell populations, in Col6a1 –/– single myofibers after 72 h culture on matrigel-coated dishes in the presence or absence of purified native collagen VI. Data are shown as mean±s.e.m. of three independent replicates (** P< 0.01; unequal variance Student’s t -test; n =10 myofibers, each group). Col VI, collagen VI; KO, Col6a1 –/– ; MG, matrigel; WT, wild-type. Full size image Table 1 Quantification of Pax7 + MyoD – , Pax7 + MyoD + and Pax7 – MyoD + cell populations on single wild type and Col6a1 –/– myofibers. Full size table Collagen VI regulates SC activity in vivo To assess whether the SC defects of collagen VI-deficient muscles may be secondary to the myopathic phenotype, we performed additional in vivo studies on Col6a1 –/– mice. Our previous work established that the myopathic phenotype of Col6a1 –/– mice is caused by a failure of the autophagic machinery in myofibers, a process that can be reinstated by feeding mice with a low-protein diet or treating them with rapamycin [8] . Based on this, we investigated whether the abnormal activity displayed by SC in Col6a1 –/– mice is secondary to the myopathic phenotype. Toward this aim, we assessed whether reactivation of autophagy in myofibers, and the consequent rescue of the myopathy, may influence the activity of Col6a1 –/– SCs. Interestingly, recovery of the autophagy-dependent myofiber defects did not exert any effect on SC activity of Col6a1 –/– mice, neither in undamaged muscles nor after cardiotoxin injury ( Supplementary Fig. S7 ). To definitely uncouple the Col6a1 –/– SC defects from the myopathy, we transplanted wild-type or Col6a1 –/– SCs into regenerating Col6a1 –/– muscle and analyzed their function in the host tissue. Indeed, if collagen VI has a direct effect on SCs in vivo , the protein expressed by transplanted wild-type cells should enable SCs to function normally in the host tissue and muscle regeneration should be significantly improved. Towards this aim, we sorted GFP + SCs derived from wild-type (WTSCs) and Col6a1 –/– (KOSCs) mice and injected them into cardiotoxin-injured Col6a1 –/– muscles ( Fig. 4a ). Real-time PCR confirmed the presence of donor WTSCs and KOSCs in host muscles and revealed expression of collagen VI in Col6a1 –/– muscles transplanted with WTSCs ( Fig. 4b ). Notably, the number of SCs in Col6a1 –/– muscles transplanted with WTSCs was significantly higher than Col6a1 –/– muscles transplanted with KOSCs ( Fig. 4d ). Concurrently, muscle regeneration was noticeably improved when Col6a1 –/– muscles were transplanted with WTSCs, compared with Col6a1 –/– muscles transplanted with KOSCs ( Fig. 4e ). These data confirm that the alterations displayed by SCs in Col6a1 –/– mice are strictly dependent on the lack of collagen VI and indicate that the production of this protein by SCs is required for their proper activity during muscle regeneration. 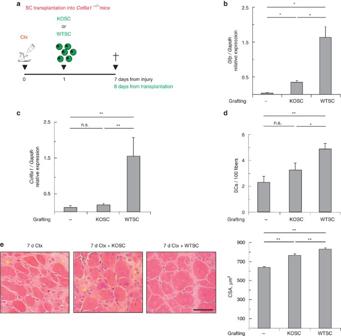Figure 4: Collagen VI has a direct effect on SCin vivo. (a) Schematic diagram of the experimental approach for grafting SCs inCol6a1–/–regenerating muscles. One day after cardiotoxin injury, 3,000 freshly isolated wild-type SCs orCol6a1–/–SCs expressing the GFP-LC3 fusion protein were injected in regeneratingCol6a1–/–TA. Muscles were analyzed after 7 days from cardiotoxin injury. (b) Real-time PCR analysis of GFP expression inCol6a1–/–muscles derived from 7-day cardiotoxin-injured mice without grafting (−) or grafted with wild-type orCol6a1–/–SCs expressing GFP-LC3. Data are shown as mean±s.e.m. of three independent replicates (*P<0.01; unequal variance Student’st-test;n=5 animals, each group). (c) Real-time PCR analysis ofCol6a1expression inCol6a1–/–muscles derived from 7-day cardiotoxin-injured mice without grafting (−) or grafted with wild-type SCs orCol6a1–/–SCs. Data are shown as mean±s.e.m. of three independent replicates (**P<0.01; n.s., not significant; unequal variance Student’st-test;n=5 animals, each group). (d) Quantification of SCs, calculated as the number of SCs on 100 fibers, inCol6a1–/–muscles derived from 7-day cardiotoxin-injured mice without grafting (−) or grafted with 3,000 wild-type SCs orCol6a1–/–SCs. Data are shown as mean±s.e.m. of three independent replicates (**P<0.01; *P<0.05; n.s., not significant; unequal variance Student’st-test;n=5–6 animals, each group). (e) Left panel, representative images of haematoxylin-eosin staining of TA cross-sections fromCol6a1–/–mice 7 days after cardiotoxin injury without grafting or grafted with wild-type SCs orCol6a1–/–SCs. The asterisks label some areas still in the degeneration phase. Scale bar, 50 μm. Right panel, quantification of myofiber mean cross-sectional area (CSA) inCol6a1–/–TA 7 days after cardiotoxin injury without grafting (−) or grafted with wild-type SCs orCol6a1–/–SCs. Data are shown as mean±s.e.m. of three independent replicates (**P<0.01; unequal variance Student’st-test;n=5–6 animals, each group). Ctx, cardiotoxin; KOSC,Col6a1–/–SCs expressing GFP-LC3 protein; WTSC, wild-type SCs expressing GFP-LC3. Figure 4: Collagen VI has a direct effect on SC in vivo. ( a ) Schematic diagram of the experimental approach for grafting SCs in Col6a1 –/– regenerating muscles. One day after cardiotoxin injury, 3,000 freshly isolated wild-type SCs or Col6a1 –/– SCs expressing the GFP-LC3 fusion protein were injected in regenerating Col6a1 –/– TA. Muscles were analyzed after 7 days from cardiotoxin injury. ( b ) Real-time PCR analysis of GFP expression in Col6a1 –/– muscles derived from 7-day cardiotoxin-injured mice without grafting (−) or grafted with wild-type or Col6a1 –/– SCs expressing GFP-LC3. Data are shown as mean±s.e.m. of three independent replicates (* P< 0.01; unequal variance Student’s t -test; n =5 animals, each group). ( c ) Real-time PCR analysis of Col6a1 expression in Col6a1 –/– muscles derived from 7-day cardiotoxin-injured mice without grafting (−) or grafted with wild-type SCs or Col6a1 –/– SCs. Data are shown as mean±s.e.m. of three independent replicates (** P< 0.01; n.s., not significant; unequal variance Student’s t -test; n =5 animals, each group). ( d ) Quantification of SCs, calculated as the number of SCs on 100 fibers, in Col6a1 –/– muscles derived from 7-day cardiotoxin-injured mice without grafting (−) or grafted with 3,000 wild-type SCs or Col6a1 –/– SCs. Data are shown as mean±s.e.m. of three independent replicates (** P< 0.01; * P< 0.05; n.s., not significant; unequal variance Student’s t -test; n =5–6 animals, each group). ( e ) Left panel, representative images of haematoxylin-eosin staining of TA cross-sections from Col6a1 –/– mice 7 days after cardiotoxin injury without grafting or grafted with wild-type SCs or Col6a1 –/– SCs. The asterisks label some areas still in the degeneration phase. Scale bar, 50 μm. Right panel, quantification of myofiber mean cross-sectional area (CSA) in Col6a1 –/– TA 7 days after cardiotoxin injury without grafting (−) or grafted with wild-type SCs or Col6a1 –/– SCs. Data are shown as mean±s.e.m. of three independent replicates (** P <0.01; unequal variance Student’s t -test; n =5–6 animals, each group). Ctx, cardiotoxin; KOSC, Col6a1 –/– SCs expressing GFP-LC3 protein; WTSC, wild-type SCs expressing GFP-LC3. Full size image Collagen VI affects SCs by regulating muscle stiffness Having established a role for collagen VI in regulating SC activity and muscle regeneration, we investigated the mechanism involved in this process. Although regulation of autophagy is a major mechanism through which collagen VI regulates myofiber homeostasis [8] , the results discussed above exclude this mechanism as a determinant for collagen VI regulation of SC activity ( Supplementary Fig. S7 ). Given the abundance of collagen VI beaded microfilaments in endomysial basement membrane [29] , we investigated whether collagen VI may be engaged in the regulation of muscle mechanical properties. Previous work demonstrated that differentiation of stem cells into myoblasts requires optimal tissue elasticity, closely matching the physiological stiffness of skeletal muscle [30] . Moreover, recent studies showed that SCs cultured on bioengineered structures mimicking muscle physiological elasticity display higher in vitro self-renewal and in vivo regeneration capabilities, when compared with cells grown on plastic [25] . To assess the contribution of collagen VI to muscle mechanical properties, we compared the stiffness of wild-type and Col6a1 –/– TA muscles using a stress–strain test. Quantification of the Young modulus, an index of elasticity, revealed that Col6a1 –/– muscles are more elastic ( E ~7 kPa) than their wild-type counterparts ( E ~12 kPa) ( Fig. 5a and Supplementary Fig. S8a ). Col6a1 –/– muscles also maintained lower stiffness 4 days after cardiotoxin injury, when there is massive ECM production, indicating that the abnormal elasticity elicited by the lack of collagen VI cannot be compensated by the increased global deposition of other ECM proteins ( Fig. 5a and Supplementary Fig. S8a ). To investigate whether the observed changes in the mechanical properties of Col6a1 –/– muscles have any major influence on in vitro SC activity, we isolated SCs from wild-type and Col6a1 –/– GFP + muscles and used them to obtain SC cultures grown on biomimetic structures with a stiffness of either ~7 kPa or ~12 kPa ( Supplementary Fig. S8b ). Wild-type SCs grown on structures of physiological (12 kPa) stiffness maintained a large proportion of Pax7 + MyoD – cells (~70% of total myogenic cells), while this proportion was dramatically decreased (<8% of total myogenic cells) when SCs were grown on structures of 7-kPa stiffness, with a corresponding increase of Pax7 + MyoD + and Pax7 − MyoD + cells ( Fig. 5b ). Notably, the total cell numbers for both wild-type and Col6a1 –/– genotypes were also markedly lower when SCs were cultured on the 7-kPa structures compared with the 12-kPa structures ( Supplementary Fig. S8c ). Altogether, this set of findings reveals that collagen VI is necessary to maintain muscle mechanical properties in vivo and that the altered stiffness displayed by Col6a1 –/– muscles affects the maintenance of Pax7 + cells in vitro . 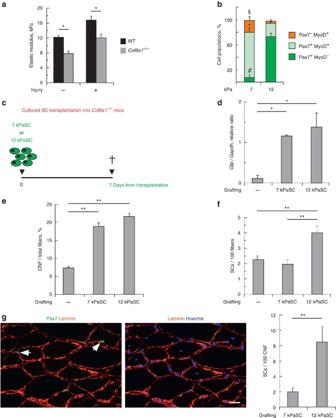Figure 5: Collagen VI affects SC self-renewal by regulating muscle stiffnessin vivo. (a) Measurement of elastic modulus of wild-type andCol6a1–/–TA muscles under standard conditions (−) and 4 days after injury (+). Data are shown as mean±s.e.m. of three independent replicates (*P<0.05; unequal variance Student’st-test;n=10 animals, each group). Error bars indicate s.d. (b) Quantification of Pax7+MyoD–, Pax7+MyoD+, and Pax7–MyoD+cell populations in sorted wild-type SCs, following 7 days culture on biomimetic structures. Data are shown as mean±s.e.m of two independent replicates (#P<0.01 for the Pax7+MyoD–population; *P<0.01 for the Pax7+MyoD+population;§P<0.01 for the Pax7–MyoD+population; unequal variance Student’st-test;n=8 wells, each group). (c) Schematic diagram of the experimental approach for grafting cultured SCs grown on 7 kPa or 12 kPa inCol6a1–/–TA muscles. (d) Real-time PCR analysis of GFP DNA content inCol6a1–/–TA under untreated condition (−) or after grafting. Data are shown as mean±s.e.m of three independent replicates (*P<0.05; unequal variance Student’st-test;n=6 animals, each group). (e) Analysis of centrally nucleated fibers (CNF) inCol6a1–/–TA under untreated condition (−) or 7 days after grafting. Data are shown as mean±s.e.m. of three independent replicates (**P<0.01; unequal variance Student’st-test;n=6 animals, each group). (f) Quantification of SCs inCol6a1–/–TA under untreated condition (−) or 7 days after grafting. Data are shown as mean±s.e.m. of three independent replicates (**P<0.01; unequal variance Student’st-test;n=6 animals, each group). (g) Left panel, representative images ofCol6a1–/–TA grafted with cultured SCs, showing SCs localized in centrally nucleated fibers (CNFs, arrows). Scale bar, 25 μm. Right panel, quantification of SCs in CNFs ofCol6a1–/–TA under untreated condition (−) or 7 days after grafting. Data are shown as mean±s.e.m. of three independent replicates (**P<0.01; unequal variance Student’st-test;n=6 animals, each group). 7 kPaSC, wild-type SCs cultured on 7 kPa; 12 kPaSC, wild-type SCs cultured on 12 kPa; Col VI, collagen VI; MG, matrigel; WT, wild-type. Figure 5: Collagen VI affects SC self-renewal by regulating muscle stiffness in vivo . ( a ) Measurement of elastic modulus of wild-type and Col6a1 –/– TA muscles under standard conditions (−) and 4 days after injury (+). Data are shown as mean±s.e.m. of three independent replicates (* P <0.05; unequal variance Student’s t -test; n =10 animals, each group). Error bars indicate s.d. ( b ) Quantification of Pax7 + MyoD – , Pax7 + MyoD + , and Pax7 – MyoD + cell populations in sorted wild-type SCs, following 7 days culture on biomimetic structures. Data are shown as mean±s.e.m of two independent replicates ( # P <0.01 for the Pax7 + MyoD – population; * P <0.01 for the Pax7 + MyoD + population; § P <0.01 for the Pax7 – MyoD + population; unequal variance Student’s t -test; n =8 wells, each group). ( c ) Schematic diagram of the experimental approach for grafting cultured SCs grown on 7 kPa or 12 kPa in Col6a1 –/– TA muscles. ( d ) Real-time PCR analysis of GFP DNA content in Col6a1 –/– TA under untreated condition (−) or after grafting. Data are shown as mean±s.e.m of three independent replicates (* P< 0.05; unequal variance Student’s t -test; n =6 animals, each group). ( e ) Analysis of centrally nucleated fibers (CNF) in Col6a1 –/– TA under untreated condition (−) or 7 days after grafting. Data are shown as mean±s.e.m. of three independent replicates (** P< 0.01; unequal variance Student’s t -test; n =6 animals, each group). ( f ) Quantification of SCs in Col6a1 –/– TA under untreated condition (−) or 7 days after grafting. Data are shown as mean±s.e.m. of three independent replicates (** P< 0.01; unequal variance Student’s t -test; n =6 animals, each group). ( g ) Left panel, representative images of Col6a1 –/– TA grafted with cultured SCs, showing SCs localized in centrally nucleated fibers (CNFs, arrows). Scale bar, 25 μm. Right panel, quantification of SCs in CNFs of Col6a1 –/– TA under untreated condition (−) or 7 days after grafting. Data are shown as mean±s.e.m. of three independent replicates (** P< 0.01; unequal variance Student’s t -test; n =6 animals, each group). 7 kPaSC, wild-type SCs cultured on 7 kPa; 12 kPaSC, wild-type SCs cultured on 12 kPa; Col VI, collagen VI; MG, matrigel; WT, wild-type. Full size image We next assessed the in vivo fate of SCs cultured on 7-kPa or 12-kPa biomimetic structures by injecting them into Col6a1 –/– TA muscles ( Fig. 5c ). The presence of donor cells in host muscles led to the induction of muscle regeneration as expected, with no significant differences between cells cultured on structures of different stiffness ( Fig. 5d ). Conversely, the number of SCs was significantly increased in muscles transplanted with SCs grown on the 12-kPa structures, but not in those transplanted with SCs grown on the 7-kPa structures ( Fig. 5f ). Interestingly, several Pax7 + cells were found in the interstitium of muscles transplanted with SCs cultured on the less stiff structures ( Supplementary Fig. S8d ), suggesting that these myogenic cells are less able to adopt a SC localization compared with SCs cultured on structures of physiological stiffness. To get a more precise evaluation of the in vivo fate of SCs, we quantified the number of SCs associated with centrally nucleated fibers and found that it was significantly higher in regenerating fibers in muscles transplanted with SCs grown on the 12-kPa structures ( Fig. 5g ). Altogether, these data indicate that SCs grown on structures mimicking the stiffness of wild-type muscle have a higher ability to preserve their stem cell function compared with SCs grown on structures mimicking the stiffness of collagen VI-deficient muscles, supporting the idea that matrix stiffness may be a key mechanism through which collagen VI exerts its effects on SCs. Collagen VI restoration rescues SC self-renewal and muscle stiffness Previous studies established that fibroblasts are the main producers of collagen VI in skeletal muscles [5] . Based on this, and with the aim to test the effect on SCs and muscle stiffness when collagen VI deposition is reinstated in Col6a1 –/– mice, we performed grafting experiments with muscle fibroblasts in TA muscles. Fibroblasts were isolated from hindlimb muscles of either wild-type (WTFB), GFP transgenic (GFPFB) or Col6a1 –/– (KOFB) mice, characterized by immunofluorescence ( Supplementary Fig. S9a ) and injected into TA muscles of Col6a1 –/– mice. Fibroblasts were found in the connective tissue of Col6a1 –/– muscles, and WTFBs, but not KOFBs, produced and secreted collagen VI ( Fig. 6a and Supplementary Fig. S9b,c ). By 4 days after injection, fibroblasts were more diffuse and collagen VI was largely localized in the endomysium nearby Pax7 + cells ( Fig. 6a and Supplementary Fig. S9b,c ). To improve collagen VI deposition and overcome the potential loss of fibroblasts by an immune reaction against GFP [31] , WTFBs or KOFBs were used and wild-type and Col6a1 –/– mice were subjected to a second graft 6 days after the initial cell injection. Collagen VI was extensively produced and deposited around myofibers of Col6a1 –/– muscles subjected to double grafting with WTFBs ( Supplementary Fig. S9d ). 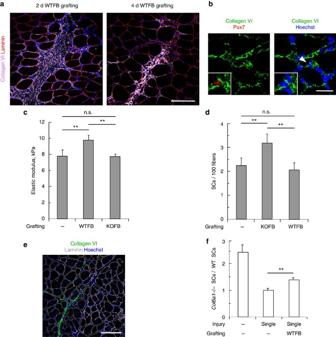Figure 6: Wild-type fibroblast grafting rescues SC self-renewal and muscle stiffness inCol6a1–/–muscles. (a) Representative confocal z-stack image of immunofluorescence analysis ofCol6a1–/–TA muscles 2 and 4 days after transplantation with wild-type fibroblasts. Sections were labeled with antibodies against collagen VI (light pink) and laminin (red). Scale bar, 100 μm. (b) Representative confocal z-stack images of immunofluorescence for collagen VI (green) and Pax7 (red) inCol6a1–/–TA sections 4 days after grafting with wild-type fibroblasts. The arrowhead points at one Pax7+cell, shown at higher magnification in the inset. Scale bar, 25 μm. (c) Quantification of the elastic modulus ofCol6a1–/–TA under untreated conditions (−) and 12 days after grafting with wild-type fibroblasts orCol6a1–/–fibroblasts. Data are shown as mean±s.d. of two independent replicates (**P<0.01; n.s., not significant; unequal variance Student’st-test;n=10 animals, each group). (d) Quantification of SCs inCol6a1–/–TA in untreated conditions (−) and in the graft region 12 days after grafting with wild-type fibroblasts orCol6a1–/–fibroblasts. Data are shown as mean±s.e.m. of three independent replicates (**P<0.01; unequal variance Student’st-test; n.s., not significant;n=6 animals, each group). (e) Representative confocal z-stack image of immunofluorescence for collagen VI (green) and laminin (gray) inCol6a1–/–TA cross-sections 30 days after injury and grafting with wild-type fibroblasts. Scale bar, 100 μm. (f) Ratio of SCs betweenCol6a1–/–and wild-type mice under untreated conditions (−) or 30 days after cardiotoxin injury either in the absence or in the presence of a single grafting with wild-type fibroblasts. Data are shown as mean±s.e.m. of three independent replicates (**P<0.01; unequal variance Student’st-test;n=6 animals, each group). Nuclei were stained with Hoechst (blue). KOFB,Col6a1–/–fibroblasts; WTFB, wild-type fibroblasts. Figure 6: Wild-type fibroblast grafting rescues SC self-renewal and muscle stiffness in Col6a1 –/– muscles. ( a ) Representative confocal z-stack image of immunofluorescence analysis of Col6a1 –/– TA muscles 2 and 4 days after transplantation with wild-type fibroblasts. Sections were labeled with antibodies against collagen VI (light pink) and laminin (red). Scale bar, 100 μm. ( b ) Representative confocal z-stack images of immunofluorescence for collagen VI (green) and Pax7 (red) in Col6a1 –/– TA sections 4 days after grafting with wild-type fibroblasts. The arrowhead points at one Pax7 + cell, shown at higher magnification in the inset. Scale bar, 25 μm. ( c ) Quantification of the elastic modulus of Col6a1 –/– TA under untreated conditions (−) and 12 days after grafting with wild-type fibroblasts or Col6a1 –/– fibroblasts. Data are shown as mean±s.d. of two independent replicates (** P <0.01; n.s., not significant; unequal variance Student’s t -test; n =10 animals, each group). ( d ) Quantification of SCs in Col6a1 –/– TA in untreated conditions (−) and in the graft region 12 days after grafting with wild-type fibroblasts or Col6a1 –/– fibroblasts. Data are shown as mean±s.e.m. of three independent replicates (** P <0.01; unequal variance Student’s t -test; n.s., not significant; n =6 animals, each group). ( e ) Representative confocal z-stack image of immunofluorescence for collagen VI (green) and laminin (gray) in Col6a1 –/– TA cross-sections 30 days after injury and grafting with wild-type fibroblasts. Scale bar, 100 μm. ( f ) Ratio of SCs between Col6a1 –/– and wild-type mice under untreated conditions (−) or 30 days after cardiotoxin injury either in the absence or in the presence of a single grafting with wild-type fibroblasts. Data are shown as mean±s.e.m. of three independent replicates (** P <0.01; unequal variance Student’s t -test; n =6 animals, each group). Nuclei were stained with Hoechst (blue). KOFB, Col6a1 –/– fibroblasts; WTFB, wild-type fibroblasts. Full size image We next investigated the effects of collagen VI deposition, by comparing wild-type and Col6a1 –/– TA muscles subjected to injection with either WTFBs or KOFBs. Notably, Col6a1 –/– TA muscles showed a significant increase of the Young modulus 12 days after grafting with WTFBs, while this physical parameter remained unchanged after grafting with KOFBs ( Fig. 6c and Supplementary Fig. S9e ). Independently from the genotype of grafted cells, injection of fibroblasts generated a response of SCs in wild-type muscles, as displayed by the local increase of centrally nucleated fibers and by the higher number of SCs ( Supplementary Fig. S10a ). Differently, the local number of SCs in Col6a1 –/– TA was increased after grafting with WTFBs, with the concurrent increase of centrally nucleated fibers, but was unaffected by grafting with KOFBs ( Fig. 6d and Supplementary Fig. S10b ). Of note, we did not observe any rescue of the SC number in areas located nearby the engraftment, but lacking collagen VI deposition, suggesting that the effects on SC activity observed in Col6a1 –/– muscles were elicited by engrafted WTFBs and collagen VI deposition, with no obvious involvement of additional cell types and/or independent paracrine mechanisms ( Supplementary Fig. S10b ). To assess whether fibroblast grafting and collagen VI deposition could also improve the maintenance of myogenic cells in Col6a1 –/– muscles after injury, WTFBs were grafted 4 h after a single cardiotoxin injection and mice were killed 30 days later. Interestingly, collagen VI was still present around Col6a1 –/– myofibers 30 days after injury ( Fig. 6e and Supplementary Fig. S10c ) and the SC ratio was significantly higher than that of the controlaterally injured non-grafted muscle, whereas no significant changes were observed in muscle weight and myofiber cross-sectional area ( Fig. 6f and Supplementary Fig. S10d,e ). Altogether, these data support a role for collagen VI in the regulation of in vivo muscle mechanical properties, which in turn can affect SC activity. The correct regulation of stem cell activity is crucial for maintaining tissue homeostasis in physiological and pathological conditions, such as after injury and during wound healing. A number of studies support the notion that the niche, a varied set of cells and extracellular factors nearby stem cells or in contact with them, has key roles in maintaining the quiescence and supporting the self-renewal of stem cells, including SCs. Our findings indicate that collagen VI, an ECM protein forming a distinctive microfibrillar system in several organs, is an essential component of muscle SC niche. A wealth of observations indicates that the ECM undergoes extensive remodeling in the course of muscle regeneration [24] . Muscle substitution by fibrotic connective tissue is a common feature of several conditions, such as aging and Duchenne muscular dystrophy, pointing at a negative effect for excessive production of fibrillar collagens and interstitial ECM components [32] . Despite this, changes of niche composition are essential for proper SC activity during muscle regeneration [19] , [24] . We found that collagen VI deposition is markedly increased during the initial phases of muscle regeneration, when the protein forms a thick network enclosing myogenic cells. Previous in vitro and in vivo studies showed that collagen VI in muscle is produced by endomysial fibroblasts, whereas neither myofibers nor myoblasts produce the protein [4] , [5] . Here, we found that collagen VI is also expressed by SCs and this expression is differently regulated during quiescence and activation. Our findings suggest that SCs are able to autoregulate the microenvironment of their niche on the basis of their behavior. Indeed, after damage, activated SCs leave their original niche for seeding in a ‘new niche’ enriched in ECM components, including collagen VI, which are mainly provided by interstitial fibroblasts. In this context, it is plausible that SCs need to change their intrinsic expression of ECM proteins, reducing the synthesis of collagen VI. Interestingly, recent literature studies support this concept by showing that SCs contribute to their own environment through the synthesis of ECM components such as collagens [33] , [34] . Moreover, it also became evident that the niche not only provides a number of molecular signals for SCs [17] , [18] , [19] , [20] , [21] , [22] , [23] , but also establishes a three-dimensional support with specific mechanical properties [10] . Healthy skeletal muscle tissue displays a definite elastic modulus ( E ~12 kPa). These biomechanical properties of muscles are altered during disease, aging and injury, as demonstrated by the stiffer elastic modulus ( E >18 kPa) of muscles of dystrophin-deficient mdx mice and of aged mice, where SC activity is compromised [10] . Our findings indicate that (i) Col6a1 –/– muscles display a distinct increase of elasticity, and that (ii) this lower stiffness is associated with a significant loss of in vitro and in vivo self-renewal capability of wild-type SCs, pointing to altered stiffness as one key mechanism underlying in vivo SC defects in collagen VI-deficient muscles. Independent evidence points to collagen VI as an ECM molecule involved in the regulation of the mechanical properties of the cell microenvironment. For instance, the pericellular matrix of articular cartilage of Col6a1 –/– mice was found to have a significantly reduced stiffness [35] , suggesting a more general biomechanical role for collagen VI in different tissues. Moreover, collagen VI null mice were shown to be resistant to genetically induced mammary tumorigenesis [36] , a process known to be particularly sensitive to the mechanical properties of the microenvironment [37] , [38] . Our findings support the concept of a strict relationship between SC homeostasis and regulation of muscle biomechanical properties ( Supplementary Fig. 11 ) [10] , [25] . Future studies, aimed at dissecting the molecular factors involved in the transduction of the mechanical signals generated by collagen VI microfilaments in muscle endomysium, will allow a more thorough understanding of the pathways through which collagen VI exerts its effects within the SC niche. Moreover, we cannot exclude possible biochemical benefits of collagen VI on SCs that might also contribute to the observed changes. Actually, such biochemical benefits are also suggested by the in vitro effects exerted by collagen VI on wild-type SCs. This scenario, together with the results obtained by transplantation experiments with different cells (freshly isolated SCs, cultured SCs and fibroblasts), suggests that collagen VI is not only important in the regulation of muscle mechanical properties, but may also provide biochemical signals to SCs. Although further studies are needed in this direction, it is intriguing to hypothesize that collagen VI could have a dual function: on one hand it is critical for the regulation of the mechanical properties of skeletal muscle, and on the other hand it may interact with some SC receptors, including those that can modulate the physical perception of the microenvironment surrounding the cells. Our study also provides new perspectives for human collagen VI diseases, as they represent non-cell-autonomous disorders of muscle [2] . The finding that cultured fibroblasts are able to secrete and deposit collagen VI in host Col6a1 –/– muscle, with beneficial effects on SCs and muscle stiffness, opens novel therapeutic venues for collagen VI-related muscular dystrophies. In various tissues, fibroblasts represent a source for collagen VI, and dermal fibroblasts derived from skin biopsies have been largely used as a diagnostic tool in patients with collagen VI mutations [3] . The possibility that fibroblasts obtained from minimally invasive biopsies may be grown in culture and used for the production and deposition of collagen VI in muscle in vivo is an attractive therapeutic option that remains to be explored in the future. Mice We performed experiments in wild-type mice of the inbred C57BL/6J strain and in Col6a1 –/– mice that we previously backcrossed in the C57BL/6J strain for eight generations [7] . We obtained data in 6-month-old mice by comparing sex-matched wild-type and Col6a1 –/– animals. We used C57BL/6J, C57BL/6-Tg(ACTB-EGFP)1Osb/J (Jackson Laboratories) and Col6a1 –/– mice to isolate muscle fibroblasts for grafting experiments. We used Col6a1 +/+ ;GFP-LC3 and Col6a1 –/– ;GFP-LC3 mice (generated in our laboratory by crossing Col6a1 –/– mice with GFP-LC3 mice [39] ) to isolate SCs for transplantation experiments. Mice were housed in individual cages in an environmentally controlled room (23 °C, 12 h light/12 h dark cycle) and provided food and water ad libitum . Native collagen VI was purified from newborn mice as previously described [7] . Mouse procedures were approved by the Ethics Committee of the University of Padova and authorized by the Italian Ministry of Health. In vivo treatments For cardiotoxin injury [27] , we anesthetized mice with isoflurane (Merial) and injected TA muscles with 30 μl cardiotoxin ( Naja mossambica mossambica , 10 μM; Sigma). Analgesia (Rimadyl) was administered for 3 days. For multiple injury experiments, TA muscles were injected with cardiotoxin 1 month after the previous injection (see also Supplementary Fig. S4C ). For cell proliferation analysis, EdU (Invitrogen) was administered for 7 days by i.p. injection at 50 mg per kg body weight every 12 h. We carried out induction of autophagy by i.p. injection with rapamycin (2 mg per kg body weight; LC Laboratories) every 24 hr for 15 days or by feeding mice with LPD (TestDiet) for 1 month [8] . For SC transplantation, we resuspended 3,000 sorted SCs in 15 μl phosphate buffered saline (PBS) and injected them into TA muscle 24 h after cardiotoxin injury. For transplantation of cultured SCs, sorted SCs were grown in culture for 1 week on biomimetic structures, then 10 4 cells were resuspended in 15 μl PBS and injected into undamaged TA muscle. For grafting with muscle fibroblasts, we resuspended 10 5 cells in 15 μl PBS and injected them into each TA muscle. For double-grafting experiments, we used the same primary culture preparation for both injections and performed the second injection 6 days after the first one. Isolation and culture of single EDL muscle fibers We carefully dissected EDL muscles from 6-month-old mice and subjected them to enzymatic digestion with collagenase I (2 mg ml −1 , Gibco) for 80 min at 37 °C. We blocked the digestion with Dulbecco’s Modified Eagle Medium (DMEM, Sigma) supplemented with 0.2 M L -glutamine (Invitrogen), 1:100 penicillin–streptomycin (Invitrogen), 1:100 fungizone (Invitrogen) and 10% horse serum (Gibco), and gently released single myofibers from muscles. With the aim to remove debris and interstitial cells, every 15–25 min, undamaged and non-contracted fibers were transferred in a new dish containing fresh medium for five times. Single selected fibers were maintained at 37 °C in a cell incubator between each wash cycle. Freshly isolated fibers were finally fixed in 4% paraformaldehyde in PBS for 15 min and maintained at 4 °C in PBS until use. For culture experiments, selected fibers were individually grown in adhesion, by placing them into chamber slides coated for at least 2 h with matrigel alone (ECM gel, Sigma) or with matrigel supplemented with purified collagen VI (5 μg cm −2 ). We cultured fibers for 72 h at 37 °C in cell incubator, using DMEM supplemented with 20% horse serum, 10% fetal bovine serum (Gibco), 1% chicken embryo extract (Sera Laboratories International) and, where indicated, 10 nM EdU (Invitrogen). Isolation and culture of SCs We dissected hindlimb muscles from mice and gently dissociated them with a MACS dissociator (Miltenyi Biotec) to yield fragmented muscle suspensions. We digested muscle suspensions for 90 min in 37 °C shaking water bath, using collagenase II (500 U ml −1 , Invitrogen) solution in Ham’s F10 medium (Sigma) supplemented with 10% horse serum (Invitrogen). We washed the fragmented myofibers and further digested them for 30 min in 37 °C shaking water bath with collagenase II (100 U ml −1 , Invitrogen) and dispase (2 U ml −1 , Invitrogen). We triturated the digested cell/fragmented fiber suspensions and washed them to yield mononucleated cell suspensions. We filtered the dissociated suspensions through 70- and 30-μm filters and labeled mononucleated cells with VCAM-biotin (1:100, 429), CD31-APC (1:100, MEC 13.3), CD45-APC (1:100, 30-F11) (all BD Bioscience) and Sca-1-Pacific-Blue (1:100, D7, Biolegend). We used streptavidin-PE-cy7 (1:100, BD Biosciences) to amplify the VCAM signal. Where indicated, single-cell preparations were labeled with anti-mouse CD31 FITC (1:100, 11-0311), anti-mouse CD45 FITC (1:100, 11-0451), anti-mouse Sca-1 FITC (1:100, 11-5981) (all eBioscence) and biotin-anti-SM/C-2.6 (1:100, a gift from S. Fukada [40] ). We used streptavidin-PerCP-Cy5.5 (1:100, BD Biosciences) to amplify the SM/C-2.6 signal. We carefully optimized cell sorting for purity and viability and subjected SM/C-2.6 + CD45 – CD31 – Sca1 – or VCAM + CD31 – CD45 – Sca-1 – cells to FACS analysis right after sorting to ensure SC purity. For culture experiments, 10 4 sorted SCs were plated on dishes coated with matrigel alone (ECM gel, Sigma) or with matrigel supplemented with purified collagen VI (5 μg cm −2 ), or on biomimetic structures coated with matrigel alone (ECM gel, Sigma). We cultured sorted SCs for 48 h or 7 days at 37 °C in cell incubator, using DMEM supplemented with 20% horse serum, 10% fetal bovine serum (Gibco), 1% chicken embryo extract (Sera Laboratories International) and, where indicated, 10 nM EdU (Invitrogen). Isolation and culture of muscle fibroblasts We used hindlimb muscles for preparing primary muscle fibroblasts by enzymatic digestion with collagenase II (100 U ml −1 , Invitrogen) and dispase (2 U ml −1 , Invitrogen) for 30 min at 37 °C. We filtered the dissociated suspensions through 70- and 30-μm filters and plated them for 10 min on gelatin-coated dishes. After removal of floating cells, we maintained the attached cells in culture until confluence. In order to enrich for fibroblasts, we expanded primary cultures for one further passage until confluence, and prepared them for cell type characterization and grafting. In vivo muscle stiffness We carefully dissected TA muscles from mice and subjected them to stress–strain tests with a Zwick/Roell Z005 device (Zwick, Germany). We anchored muscles to the jaws of the device using a suture thread, and subjected them to two consecutive compressive load–unload cycles with the following settings: 0.01 mm s −1 , strain rate; 10% strain, end of loading phase (compared with the initial sample length); no load, end of load–unload cycle. We calculated the elastic modulus from the first linear portion of the stress–strain curve for each cycle. Biomimetic structures For the generation of biomimetic structures, we prepared a solution of 3% ( w / v ) gelatin (Sigma) in PBS or of 5% ( w / v ) gelatin in PBS. Genipin (Challenge Bioproducts Co., Ltd) was added to the solutions at 0.2% ( w / w ). Each mixture was kept at 40 °C under moderate stirring, until polymerization was completed as indicated by turning into blue color. Samples were left drying at room temperature for 48 h, rinsed in water to remove genipin residues, sterilized under UV light and then kept in PBS until use at 4 °C. The mechanical properties of genipin-crosslinked biomimetic structures were measured with a Zwick/Roell Z005 device. Samples were subjected to compressive load–unload cycles with the following settings parameters: 0.01 mm s −1 , strain rate; 10% strain, end of loading phase; no load, end of load–unload cycle. The Young’s modulus of each sample was evaluated from the slope of the initial linear portion of the stress–strain curve. Biomimetic structures composed by 3% gelatin were characterized by an elastic modulus of ~7 kPa, whereas those composed by 5% gelatin displayed an elastic modulus of ~12 kPa. At least three specimens for each composition were tested. Biomimetic structures were maintained in culture medium at 37 °C overnight, before SC plating. Statistical analyses We expressed data as means±s.e.m. or, where indicated, as means±s.d. We determined statistical significance by unequal variance Student’s t -test. A P -value<0.05 was considered statistically significant. Other methods Additional information on methods is provided in Supplementary Methods . How to cite this article: Urciuolo, A. et al. Collagen VI regulates satellite cell self-renewal and muscle regeneration. Nat. Commun. 4:1964 doi: 10.1038/ncomms2964 (2013).